Reconstitution of a nanomachine driving the assembly of proteins into bacterial outer membranes In biological membranes, various protein secretion devices function as nanomachines, and measuring the internal movements of their component parts is a major technological challenge. The translocation and assembly module (TAM) is a nanomachine required for virulence of bacterial pathogens. We have reconstituted a membrane containing the TAM onto a gold surface for characterization by quartz crystal microbalance with dissipation (QCM-D) and magnetic contrast neutron reflectrometry (MCNR). The MCNR studies provided structural resolution down to 1 Å, enabling accurate measurement of protein domains projecting from the membrane layer. Here we show that dynamic movements within the TamA component of the TAM are initiated in the presence of a substrate protein, Ag43, and that these movements recapitulate an initial stage in membrane protein assembly. The reconstituted system provides a powerful new means to study molecular movements in biological membranes, and the technology is widely applicable to studying the dynamics of diverse cellular nanomachines. The vast majority of proteins in the outer membrane of pathogenic bacteria have a β-barrel architecture, and how such proteins are assembled remains an important question in biology. The assembly pathway for these outer membrane proteins is highly conserved in bacteria [1] ; this essential cellular pathway depends on a set of factors that select and assist protein substrates en route to the outer membrane [1] , [2] , [3] , [4] , [5] , [6] . A network of periplasmic chaperones and proteases serve quality-control functions in the pathway (for example, Skp and DegP) [7] , [8] , [9] , [10] , [11] , [12] , [13] and molecular chaperones such as SurA also assist the loading of the nascent membrane protein substrates onto the face of the outer membrane [14] , [15] , [16] , [17] . The essential protein BamA can be purified from outer membranes of Escherichia coli (E. coli) as a hetero-oligomeric BAM (β-barrel assembly machinery) complex, associated tightly with the lipoproteins: BamB, BamC, BamD and BamE [14] , [18] , [19] , [20] . The BAM complex and a further module of the BAM, the translocation and assembly module (TAM), catalyse the insertion and assembly of nascent membrane proteins into the plane of the outer membrane [1] , [2] , [3] , [4] , [5] . The TAM is a nanomachine composed of two proteins: the outer membrane protein TamA and the TamB subunit, anchored to the inner membrane [21] . TamA is a member of the Omp85/FhaC superfamily of proteins [22] , with a characteristic β-barrel domain in the plane of the outer membrane, as well as three POTRA domains that sit within the periplasm [21] , [23] . The crystal structure of TamA revealed a crucial incomplete matching in the first and last β-strand in the membrane-embedded domain, which was proposed to assist substrate protein assembly [23] . TamB has an amino-terminal signal-anchor sequence integrated in the inner membrane, with the vast bulk of TamB predicted to be β-helical in structure, and contained within the periplasm [21] , [24] , [25] , [26] . An interaction of the POTRA domain of TamA to TamB stabilizes the interaction between these two protein subunits, and the TAM can therefore be purified from detergent-solubilized membranes using immunoprecipitation or blue-native polyacrylamide gel electrophoresis (BN–PAGE) [21] . The precise function of the TAM in the β-barrel assembly pathway has been difficult to dissect in complex cellular systems, a problem often encountered in the study of membrane-located nanomachines. Here we sought to develop a system to study the movement and activity of the TAM. To this end, TamA and TamB were purified and reconstituted into a membrane environment suitable for interrogation by magnetic contrast neutron reflectrometry (MCNR). MCNR systems employ an internal reference layer to enhance the resolution of the measurement [27] , [28] , [29] , and these systems excel at interrogating fully hydrated soft matter on atomically flat gold surfaces. We therefore reasoned that MCNR could be an exciting new means to measure movements in nanomachines within a membrane layer, provided a membrane of sufficient quality could be reconstituted. The TAM was reconstituted into a membrane on a nickel-NTA ( N α , N α -bis-(carboxymethyl)- L -lysine) functionalized gold surface, for characterization by quartz crystal microbalance with dissipation (QCM-D) and MCNR. The MCNR studies provided structural resolution down to 1 Å, enabling accurate measurement of protein domains projecting from the phospholipid bilayer of the membrane. These measurements reconcile well with the dimensions in the recent crystal structure of TamA and with atomic force microscopy (AFM) and dynamic light scattering measurements of TamB. We show that movements of TamA within the TAM are initiated in the presence of a substrate protein, Ag43. These movements recapitulate an initial stage in membrane protein assembly, and Ag43 was observed to enter the membrane layer in MCNR experiments. This reconstituted system reports on the function of the TAM and provides a powerful new means to study molecular movements in biological membranes, with the technology applicable to studying the dynamics of diverse cellular nanomachines. Reconstitution of the TAM in a planar lipid environment These studies required TamA to be attached to an engineered gold surface. Informed by the crystal structure of TamA [23] ( Supplementary Fig. 1a ), a metal-binding sequence comprising six histidine residues (His 6 ) was engineered into an extracellular loop of TamA ( Fig. 1a and Supplementary Fig. 1b ). This His 6 modification of TamA does not affect the integrity of the TAM, as judged by the co-immunoprecipitation of TamA with TamB ( Fig. 1b ), and by co-purification of TamA with TamB by BN–PAGE ( Fig. 1c ). The modified loop is exposed on the extracellular surface, as anti-His 6 antibodies can be used to decorate intact E. coli cells expressing this form of TamA ( Fig. 1d and Supplementary Fig. 1c ). 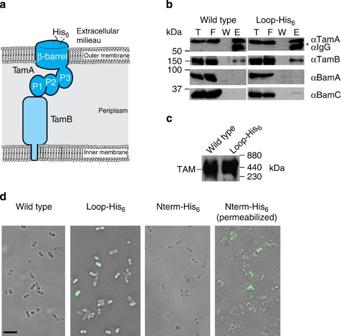Figure 1: Insertion of a His6 sequence into an external loop of TamA. (a) Topology of TamA: a β-barrel domain embedded in the outer membrane and three POTRA domains (P1, P2 and P3) exposed to the periplasm of the bacterial cell. Orientation of the nickel-binding sequence (His6) is shown. (b) Membrane extracts prepared fromE. coliexpressing TamA (wild type) or TamA with ‘loop-His6’ sequence (Supplementary Fig. 1), were subject to immunoprecipitation with the anti-TamA and Protein A-Sepharose, followed by detection with the indicated antibodies after SDS–PAGE.T, 10% of the total proteins;F, 10% of the flow-through fraction;W, 20% of the last three wash fraction;E, 100% of the eluted proteins. (c) Alternatively, to assess interaction of TamA and TamB subunits as the ~440 kDa TAM, membrane extracts prepared fromE. coliexpressing either TamA or the loop-His6form of TamA, were analysed by BN–PAGE and immunoblotting. (d)E. coliexpressing TamA (wild-type) without a His6sequence, TamA with the loop-His6epitope or the control N-terminal N-His6-epitope (as documented inSupplementary Fig. 1) were subject to immunofluorescence microscopy. A second sample of cells was permeabilized to provide access to the periplasm for immunostaining. Scale bar, 10 μm. Figure 1: Insertion of a His6 sequence into an external loop of TamA. ( a ) Topology of TamA: a β-barrel domain embedded in the outer membrane and three POTRA domains (P1, P2 and P3) exposed to the periplasm of the bacterial cell. Orientation of the nickel-binding sequence (His 6 ) is shown. ( b ) Membrane extracts prepared from E. coli expressing TamA (wild type) or TamA with ‘loop-His 6 ’ sequence ( Supplementary Fig. 1 ), were subject to immunoprecipitation with the anti-TamA and Protein A-Sepharose, followed by detection with the indicated antibodies after SDS–PAGE. T , 10% of the total proteins; F , 10% of the flow-through fraction; W , 20% of the last three wash fraction; E , 100% of the eluted proteins. ( c ) Alternatively, to assess interaction of TamA and TamB subunits as the ~440 kDa TAM, membrane extracts prepared from E. coli expressing either TamA or the loop-His 6 form of TamA, were analysed by BN–PAGE and immunoblotting. ( d ) E. coli expressing TamA (wild-type) without a His 6 sequence, TamA with the loop-His 6 epitope or the control N-terminal N-His 6 -epitope (as documented in Supplementary Fig. 1 ) were subject to immunofluorescence microscopy. A second sample of cells was permeabilized to provide access to the periplasm for immunostaining. Scale bar, 10 μm. Full size image Reconstitution of TamA within a synthetic membrane was achieved using a gold-coated, near atomically flat silicon wafer functionalized with NTA ( Supplementary Fig. 2 ), with nickel ions creating a nickel-NTA-functionalized gold surface. QCM-D was used for proof-of-principle measurements to assess the deposition of protein and lipid on the surface. In QCM-D, temporal changes in frequency (Δ f ) and dissipation (Δ D ) reflect the mass and viscoelasticity of the surfaces, respectively [30] , [31] , [32] . Measurements showed a frequency decrease corresponding to the mass uptake on the sensor surface caused by detergent-solubilized TamA ( Fig. 2a , step 1). After washing the nickel-NTA:TamA:detergent surface ( Fig. 2a , step 2), a supported membrane was formed by phospholipid adsorption, displacing the detergent ( Fig. 2a , step 3) [33] . To extend these findings, we then reconstituted the TAM nanomachine by addition of TamB. A truncated form of TamB was engineered to lack key residues in the N-terminal signal-anchor sequence that retains it in the inner membrane ( Fig. 2b ); this TamB(ΔTM) was thereby expressed as a soluble protein in the periplasm of E. coli and purified in soluble form. A proportion of TamB(ΔTM) associates with TamA to form a TAM complex ( Fig. 2c ), with the BN–PAGE analysis revealing an increase in faster-migrating forms of TamA that might represent monomers or homodimers not associated with TamB. TamB(ΔTM) purified from the periplasm by affinity chromatography and size-exclusion chromatography was thereafter used to reconstitute the TAM in QCM-D experiments. 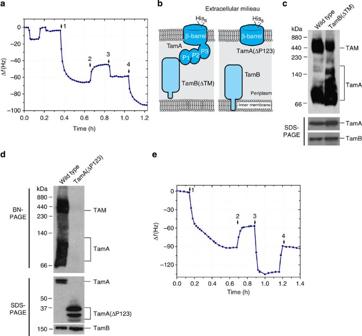Figure 2: A synthetic membrane incorporating the outer membrane protein TamA. (a) QCM-D measurements show the frequency response, indicative of mass changes, to (1) the attachment of TamA to the gold surface, (2) washing away of detergent with a positive frequency shift, (3) reconstitution of the membrane layer with phospholipids, followed by rinsing att=0.95 h and (4) the addition of purified TamB revealing a frequency response of ~30 Hz. (b) Schematic summary of TamA and TamB constructs used in QCM-D analysis. (c) Membrane extracts fromE. coliexpressing thetamABoperon, or a modifiedtamABoperon that expresses TamBΔTM, were analysed by BN–PAGE followed by immunoblotting for TamA. Samples of each extract were assessed in parallel by SDS–PAGE (lower panel) to determine the relative level of TamA and TamB/TamBΔTM in each extract. (d) Total membranes fromE. coliexpressing thetamABoperon (containing wild-type TamA-His6) or a modifiedtamABoperon (containing TamAΔP123-His6) were analysed by BN–PAGE and immunoblotting (upper panel) to assess the formation of the TAM, and SDS–PAGE and immunoblotting (bottom panel) to determine the relative level of TamA/ TamAΔP123 and TamB in each extract. (e) QCM-D measurements show the frequency response, indicative of mass changes, for membranes reconstituted from TamA(ΔP123). (1) Detergent-solubilized TamA(ΔP123) was added to the gold surface, (2) washing of detergent with positive frequency change and (3) reconstitution of the membrane layer after addition of POPC, followed by rinsing away unbound POPC att=1 h, revealing a positive frequency change, and (4) the addition of TamB indicating no binding to TamA(ΔP123). Figure 2: A synthetic membrane incorporating the outer membrane protein TamA. ( a ) QCM-D measurements show the frequency response, indicative of mass changes, to (1) the attachment of TamA to the gold surface, (2) washing away of detergent with a positive frequency shift, (3) reconstitution of the membrane layer with phospholipids, followed by rinsing at t =0.95 h and (4) the addition of purified TamB revealing a frequency response of ~30 Hz. ( b ) Schematic summary of TamA and TamB constructs used in QCM-D analysis. ( c ) Membrane extracts from E. coli expressing the tamAB operon, or a modified tamAB operon that expresses TamBΔTM, were analysed by BN–PAGE followed by immunoblotting for TamA. Samples of each extract were assessed in parallel by SDS–PAGE (lower panel) to determine the relative level of TamA and TamB/TamBΔTM in each extract. ( d ) Total membranes from E. coli expressing the tamAB operon (containing wild-type TamA-His 6 ) or a modified tamAB operon (containing TamAΔP123-His 6 ) were analysed by BN–PAGE and immunoblotting (upper panel) to assess the formation of the TAM, and SDS–PAGE and immunoblotting (bottom panel) to determine the relative level of TamA/ TamAΔP123 and TamB in each extract. ( e ) QCM-D measurements show the frequency response, indicative of mass changes, for membranes reconstituted from TamA(ΔP123). (1) Detergent-solubilized TamA(ΔP123) was added to the gold surface, (2) washing of detergent with positive frequency change and (3) reconstitution of the membrane layer after addition of POPC, followed by rinsing away unbound POPC at t =1 h, revealing a positive frequency change, and (4) the addition of TamB indicating no binding to TamA(ΔP123). Full size image Addition of purified TamB to the TamA membrane resulted in a decrease in frequency of ~95 Hz ( Fig. 2a , step 4), reflecting the greater mass of the TAM (that is, TamA+TamB) relative to the TamA subunit alone. To be certain that this docking of TamB to the membrane was a specific reconstitution of the TAM rather than a nonspecific affinity between TamB and the lipid component of the membrane, a new construct was designed wherein the three POTRA domains of TamA were deleted ( Fig. 2b ). Expressed in E. coli , this TamA(ΔP123) truncated protein fails to bind TamB as judged by BN–PAGE ( Fig. 2d ). In QCM-D experiments, the TamA(ΔP123) behaves as per the intact TamA protein: measurements showed a frequency decrease corresponding to the mass uptake for detergent-solubilized TamA(ΔP123) ( Fig. 2e , step 1) and, after washing the surface ( Fig. 2e , step 2), a supported membrane was formed by phospholipid adsorption, displacing the detergent ( Fig. 2e , step 3). Importantly, no binding event was observed when TamB was added to the membrane containing TamA(ΔP123) ( Fig. 2e , step 4). Defining the membrane with neutron reflectrometry For MCNR analysis, single crystal silicon blocks polished on one face were coated by electron beam deposition with an ~44 Å layer of magnetic alloy followed by ~170 Å of gold. This gold-coated surface was in turn functionalized with nickel-NTA using the procedure we developed ( Supplementary Fig. 2 ). Before attaching the membrane layer, the NTA layer on the gold surface was characterized with two different magnetic contrasts and two water contrasts (D 2 O and H 2 O) ( Supplementary Fig. 3 ), with the thickness of the NTA layer thereby determined to be 17±1 Å. TamA was added onto the nickel-NTA-modified surface, followed by the addition of lipids for membrane reconstitution. MCNR measurements were indicative of TamA binding to the surface ( Supplementary Fig. 4 ) and showed a membrane layer was formed ( Supplementary Fig. 5 ). Isotopic contrasting (that is, with D 2 O, H 2 O or a mixture thereof) enabled experiments in which a specific protein component, or the lipid of the membrane system, could be selectively visualized. Magnetic and isotopic contrasting yielded data analysed using an optical matrix method [27] , [28] ; in this way the surface is considered to be made up of discrete layers extending uniformly in a lateral direction, with a constant thickness and scattering length density (SLD). Reflection and transmission occur at each interface where there is a change of SLD ( Fig. 3a ), and the total signal consists of the summation of contributions from each interface. 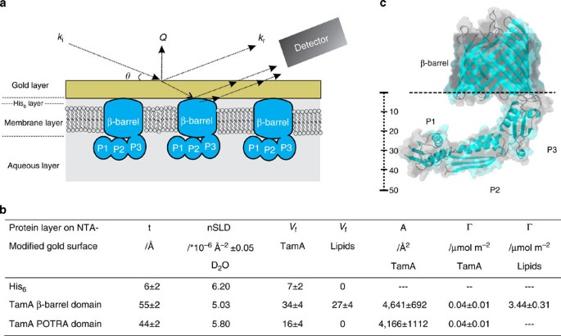Figure 3: Structure of TamA in the membrane environment. (a) In the MCNR experimental system, neutrons probe the molecular structure attached to the gold surface, including components of the membrane layer and projections into the aqueous layer.kirepresents the incident neutron beam,krthe reflected beam,θthe incident and exit angles of the neutron beam andQdenotes the scattering vector. (b) The volume fraction (Vf) of both the TamA membrane-embedded (β-barrel) domain, and the POTRA domains in the aqueous layer, as derived from six contrasts (Supplementary Fig. 4b). Assembly of membrane around the TamA β-barrel domain is shown inSupplementary Fig. 5. t, thickness; nSLD, scattering length density;Vf, volume fraction; A, area per molecular; Γ, surface excess. Where applicable, ±denotes the s.d. (c) Crystal structure of TamA23(pdb P0ADE4), highlighting the molecular dimensions of the POTRA domains P1, P2 and P3. Figure 3: Structure of TamA in the membrane environment. ( a ) In the MCNR experimental system, neutrons probe the molecular structure attached to the gold surface, including components of the membrane layer and projections into the aqueous layer. k i represents the incident neutron beam, k r the reflected beam, θ the incident and exit angles of the neutron beam and Q denotes the scattering vector. ( b ) The volume fraction ( V f ) of both the TamA membrane-embedded (β-barrel) domain, and the POTRA domains in the aqueous layer, as derived from six contrasts ( Supplementary Fig. 4b ). Assembly of membrane around the TamA β-barrel domain is shown in Supplementary Fig. 5 . t, thickness; nSLD, scattering length density; V f , volume fraction; A, area per molecular; Γ, surface excess. Where applicable, ±denotes the s.d. ( c ) Crystal structure of TamA [23] (pdb P0ADE4), highlighting the molecular dimensions of the POTRA domains P1, P2 and P3. Full size image For the purposes of data fitting, TamA was separated into three sublayers: a His 6 extramembrane layer, a membrane layer (containing the β-barrel domain of TamA) and an aqueous layer (which includes the POTRA domain of TamA) ( Fig. 3b and Supplementary Fig. 4 ). The data showed a hydrated hexa-histidine layer of 6±2 Å containing at least 90% water, and the thickness measured for the β-barrel domain of TamA is 55±2 Å. TamA has an area per molecule of 4,641 Å 2 , with a volume fraction ( V f ) of 34% ( Fig. 3b and Supplementary Fig. 4c ). The POTRA domains of TamA project 44±2 Å into the aqueous layer, relative to the internal face of the combined membrane layer ( Fig. 3b ) in agreement with observations from the crystal structure of TamA [23] ( Fig. 3c ). With the addition of lipids to reconstitute a membrane environment, reflectivity profiles shifted characteristically, demonstrating the assembly of a membrane layer on the surface ( Supplementary Fig. 5a ). As a result, the SLD in the β-barrel domain decreased from 5.70 × 10 −6 to 5.03 × 10 −6 Å −2 , while the SLD of the POTRA domains in the aqueous layer remained the same. SLD measurements reflect changes of atomic composition and density; the data gathered are consistent with the expectation that phospholipid fills the gap between the TamA molecules, corresponding to a coverage of 27±4% of the experimental surface ( Fig. 3b and Supplementary Fig. 5c ). Architecture of TamA and TamB within the TAM MCNR was then used to determine the orientation of the TamB subunit in the reconstituted TAM. Addition of TamB did not change the physical environment (or SLD) of TamA ( Fig. 4a and Supplementary Fig. 6 ). The fitted data from three different water contrasts (that is, with either D 2 O, H 2 O or a mixture thereof) and two magnetic contrasts showed that addition of TamB results in a protein projection from the membrane of ~200 Å ( Supplementary Fig. 6 ). The SLDs corresponding to the 44 Å projection of the POTRA domains of TamA do not change, suggesting that TamB provides a ~160 Å extension of the TAM into the aqueous layer ( Fig. 4a ). This is consistent with previous secondary structure and tertiary structure modelling of TamB, which had proposed an elongate, β-helical structure [24] , [25] , [26] akin to those seen in haemagluttinins and autotransporter passenger domains ( Fig. 4b ). Dynamic light scattering ( Fig. 4c ) provided direct measurements of the soluble TamB, with the calculated size of TamB having a hydrodynamic radius of 174 Å, with a monodisperse size distribution (polydispersity index of ~0.17). Measurements using AFM support this, with TamB observed as an elongated shape, with a molecular height of 20 Å and length of 160 Å ( Fig. 4d ). Taking the AFM, light scattering and MCNR measurements together, we conclude that TamB is an elongated molecule and stands end-on perpendicular to the membrane, contacting the POTRA domains of TamA ( Fig. 4e ). 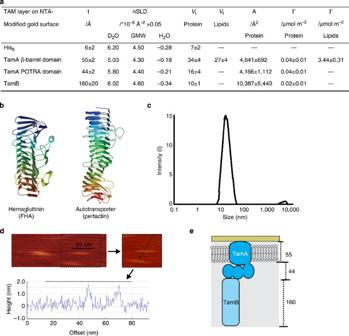Figure 4: Reconstitution of the TAM. (a) Fitted MCNR data measurements of TamB docking to the TamA layer: the volume fraction (Vf) of both TamA β-barrel and POTRA domains are derived from six contrasts (Supplementary Fig. 5). After addition of TamB, further measurements made are detailed inSupplementary Fig. 6. The parameters of the reconstituted TAM are calculated using six contrasts. t, thickness; nSLD, scattering length density;Vf, volume fraction; A, area per molecular; Γ, surface excess. Where indicated, ±denotes the s.d. (b) Structures of two β-helical bacterial proteins, the haemagglutinin FHA (pdb code 1RWR) and the passenger domain of the autotransporter pertactin (pdb code 1DAB). (c) Dynamic light scattering result for the soluble preparation of TamB. (d) Solution AFM imaging of TamB on a mica surface (scale bar, 20 nm). Cross-sectional data corresponding to the dashed line is shown below the images. (e) Pictorial representation of the TAM based on MCNR and AFM data. Figure 4: Reconstitution of the TAM. ( a ) Fitted MCNR data measurements of TamB docking to the TamA layer: the volume fraction ( V f ) of both TamA β-barrel and POTRA domains are derived from six contrasts ( Supplementary Fig. 5 ). After addition of TamB, further measurements made are detailed in Supplementary Fig. 6 . The parameters of the reconstituted TAM are calculated using six contrasts. t, thickness; nSLD, scattering length density; V f , volume fraction; A, area per molecular; Γ, surface excess. Where indicated, ±denotes the s.d. ( b ) Structures of two β-helical bacterial proteins, the haemagglutinin FHA (pdb code 1RWR) and the passenger domain of the autotransporter pertactin (pdb code 1DAB). ( c ) Dynamic light scattering result for the soluble preparation of TamB. ( d ) Solution AFM imaging of TamB on a mica surface (scale bar, 20 nm). Cross-sectional data corresponding to the dashed line is shown below the images. ( e ) Pictorial representation of the TAM based on MCNR and AFM data. Full size image Substrate-induced movements of the TAM Having reconstituted the TAM nanomachine, we sought to understand how the machine behaves when it encounters a substrate protein. In vivo , the efficient assembly of the β-barrel protein Ag43 depends on the TAM [21] . Urea-denatured Ag43 was purified ( Supplementary Fig. 7a ) to address its interactions with the supported membrane. QCM-D measurements confirmed there was no significant association of Ag43 with the membrane observed in the absence of the TAM ( Supplementary Fig. 7b ), or in the presence of TamA(ΔP123) ( Supplementary Fig. 7c ). However, when Ag43 was added to the reconstituted TAM, the reflectivity curve shifted ( Fig. 5a and Supplementary Fig. 7d ) and data from magnetic and solvent contrast experiments ( Supplementary Fig. 7e ) indicated a concomitant movement of POTRA domains of TamA, such that they come to project 77 Å away from the membrane surface. Within the membrane layer, selective isotopic labelling allows the contribution of lipid and Ag43 and the β-barrel domain of TamA to be calculated (using the equation ρ = φ A ρ A + φ B ρ B + φ w ρ w ; see Methods). The values thus derived for Ag43 and phospholipids showed that the volume fraction of phospholipid in the membrane layer decreased greatly from ~27%, with a concomitant appearance of Ag43 (from 0 to a volume fraction of ~11%) in the membrane layer ( Fig.5b and Supplementary Fig. 7f ). This displacement of lipid by Ag43 is likely to be a consequence of the physical constraints of the experimental system; in vivo , the lipids could move laterally to accommodate the protein mass of the inserted Ag43. 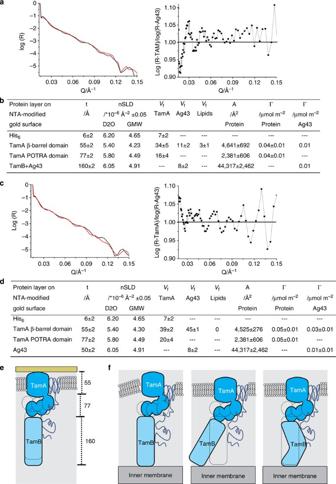Figure 5: Dynamics of the TAM measured in response to substrate binding. (a) MCNR curves of the TAM with addition of Ag43 (left panel): responses before addition of Ag43 (black) and after addition of Ag43 (red). To document the impact of the addition of Ag43, the ratio of the reflectivity curve changes (right panel) use log(R-TAM)/log(R-TAM+Ag43) as a function ofQ.Supplementary Fig. 7documents the data acquisition and calculations. (b) Table of the fitted and calculated parameters after addition of Ag43 to the TAM. Where applicable, ±denotes the s.d. (c) MCNR curves of TamA with addition of Ag43 (left panel): responses before addition of Ag43 (black) and after addition of Ag43 (red). The ratio of the reflectivity curve changes (right panel) use log(R-TamA)/log(R-TamA+Ag43) as a function ofQandSupplementary Fig. 8details the data acquisition and calculations. (d) Table of the fitted and calculated parameters after addition of Ag43 to TamA. Where indicated, ±denotes the s.d. (e) Pictorial representation summarizing movements of the TAM seen in the MCNR experimental system. (f) With the spatial constraints of the inner membrane as would occurin vivo, movements of TamB would either deform the membrane layer, or act to laterally shift TamA relative to TamB, or deform the TamB subunit. Figure 5: Dynamics of the TAM measured in response to substrate binding. ( a ) MCNR curves of the TAM with addition of Ag43 (left panel): responses before addition of Ag43 (black) and after addition of Ag43 (red). To document the impact of the addition of Ag43, the ratio of the reflectivity curve changes (right panel) use log(R-TAM)/log(R-TAM+Ag43) as a function of Q . Supplementary Fig. 7 documents the data acquisition and calculations. ( b ) Table of the fitted and calculated parameters after addition of Ag43 to the TAM. Where applicable, ±denotes the s.d. ( c ) MCNR curves of TamA with addition of Ag43 (left panel): responses before addition of Ag43 (black) and after addition of Ag43 (red). The ratio of the reflectivity curve changes (right panel) use log(R-TamA)/log(R-TamA+Ag43) as a function of Q and Supplementary Fig. 8 details the data acquisition and calculations. ( d ) Table of the fitted and calculated parameters after addition of Ag43 to TamA. Where indicated, ±denotes the s.d. ( e ) Pictorial representation summarizing movements of the TAM seen in the MCNR experimental system. ( f ) With the spatial constraints of the inner membrane as would occur in vivo , movements of TamB would either deform the membrane layer, or act to laterally shift TamA relative to TamB, or deform the TamB subunit. Full size image To specifically address the role of TamA in Ag43 assembly, we analysed the behaviour of Ag43 in the absence of TamB ( Supplementary Fig. 8 ). Differences in the reflectivity curves in the values corresponding to the critical edge (at Q =0.01–0.03 Å −1 ) suggest significant structural changes on adding Ag43, consistent with a binding event ( Fig. 5c ). The SLD values for the membrane-embedded domain of TamA ( Fig. 5d and Supplementary Fig. 8c ) demonstrate the accumulation of Ag43 in the membrane layer. The volume fraction calculations demonstrate that with TamA alone, the volume fraction of Ag43 in the membrane layer increased to 45%. The surface excess of Ag43, a reflection of the amount of Ag43 bound to the membrane, was found to be three times more than the value achieved with the complete TAM nanomachine ( Fig. 5d ). We conclude that TamA is necessary and sufficient to initiate the penetration of Ag43 into a membrane layer, and that TamB regulates this activity of TamA. In summary, the fitted MCNR data demonstrates that in the presence of Ag43, the POTRA domain of TamA changes conformation to project 77 Å out from the membrane surface ( Fig. 5e ). In a cellular context, the N terminus of TamB is anchored into the inner membrane [21] , and the inner membrane is rigidified through turgor pressure [34] ; hence, such movements of TamA would either deform the outer membrane or change the disposition of TamB within the nanomachine: tilting TamB if it is a rigid body, or bending TamB if the molecule has flexibility ( Fig. 5f ). The force exerted on TamB in any of these molecular scenarios would provide a basis for the nanomachine to reset the starting conformation in TamA, after completion of a protein assembly event in the bacterial outer membrane. Protein targeting and assembly pathways are fundamental aspects of cell biology, but the nanomachinery that drive them are often refractory to direct analysis. MCNR analysis here has shown that a membrane-embedded nanomachine can be reconstituted in a system amenable to direct observation on how it reacts to a substrate protein. As selective deuterium-based labelling allows specific measurement of each protein component and the phospholipid layer of the reconstituted membrane system, and because the technique is reliable down to 1 Å measurements, MCNR enables a highly precise and insightful characterization of nanomachines such as the TAM. This study demonstrates that MCNR is a powerful new means to characterize molecular movements in membrane proteins, and this technology is widely applicable to understanding the function of nanomachines that operate in diverse cellular processes. Materials General reagents were purchased from Sigma-Aldrich unless otherwise stated. 1-palmitoyl-2-oleoyl- sn -glycero-3-phosphocholine (POPC), 1-palmitoyl (d31)-2-oleoyl- sn -glycero-3-phosphocholine and n-dodecyl β- D -maltoside (DDM) were from Avanti Polar Lipids, Inc. Elugent, 50% solution was purchased from Calbiochem. These chemicals were used as received without further purification. Polished silicon blocks were purchased from Crystran Ltd (Poole, Dorset, UK). Bacterial strains The E. coli strains used for functional analysis of the His 6 -modified TamA were BW25113, BW25113 tamA :: kan and BW25113 tamB :: kan [35] . Removal of the antibiotic-resistant marker to create BW25113 Δ tamA and BW25113 Δ tamB was done so using plasmid pCP20 (ref. 36 ). A BW25113 Δ tamAB mutant was used for expression of the modified tamAB operon expressing the TamBΔTM or TamAΔP123 plasmid constructs. For overexpression and purification of TamA, TamB and Ag43, the host E. coli strain TOP10 was used. Plasmid construction A codon-optimized tamAB gene was synthesized de novo by GenScript and cloned into pBADHisA (Invitrogen, UK) to generate pBADTamAB. A 365-bp Kpn I- Ngo MIV fragment comprising the end of tamA and the start of tamB with a hexahistidine-tag inserted into the coding region corresponding to the eighth interstrand loop (Loop 8) of TamA was synthesized de novo and cloned into pUC57 (GenScript). pUC57TamAB-C-term-6xHis was digested with Kpn I and Ngo MIV, and subcloned into pBADTamAB, predigested with the same restriction enzymes to generate pBADTamAB-C-term-6xHis. To construct TamAΔP123, a 437-bp fragment was synthesized de novo and cloned into pUC57. pUC57TamABΔP123 was digested separately with Mlu I and Eco RI, Mlu I and Bst BI, and with Mlu I and Spe I, and subcloned into pBADTamAB-C-term-6xHis, predigested with the same restriction enzymes, to create pBADTamAB-C-term-6xHisΔP123. To construct pBADTamABΔTM-C-term-6xHis, a hexahistidine-tagged form of TamB with a truncated signal-anchor sequence (ΔL 16 -L 25 ), megaprimer PCR was performed as described previously [37] , with some variation. Briefly, a round 1 PCR was performed on 500 ng of template DNA (pBADTamAB-C-term-6xHis) with 1 μg of mutagenesis primer TamBΔTM15 (5′-CAGCCTCGGCGTGGTTATCGTTATCGGTGGTGGCGTGGGCACCACCAGCGGCCTGCATC-3′) in combination with 1 μg of primer TamABNgoMIVRev (5′-ATTGCCGGCTTTTACCGC-3′) per 100 μl of reaction mixture. The round 1 PCR was then purified to remove residual primers from the megaprimer synthesized in this first round of amplification. A round 2 PCR was performed with 4 μg of megaprimer and 1 μg of primer TamABKpnIFor (5′-CGGGTACCGGGGTCGG-3′) on 500 ng of template DNA (pBADTamAB-C-term-6xHis) per 100 μl of reaction mixture. The round 2 amplicon and target vector (pBADTamAB-C-term-6xHis) were then digested with Kpn I and Ngo MIV, and ligated. To construct pBADTamA-C-term-6xHis, pBADTamA-C-term-6xHisΔP1-3, PCR was performed on 500 ng of template DNA (pBADTamAB-C-term-6xHis) with 1 μg each of primers TamA Mlu IFor (5′-GAAACGCGTAACAAAAGTGTCTATAATCACG-3′) and TamA Hind IIIRev (5′-CAGCCAAGCTTTCATAATTCTGGCCCCAGA-3′). Amplicons and target vector (pBADHisA) were then digested with Mlu I and Hind III, and ligated. Immunofluorescence immunoprecipitation and immunoblotting TOP10 tamAB::kan E. coli cells transformed with pBADTamAB (wild type) and pBADTamABHis6 (TamAB loop-His6) were grown to mid-log phase in 0.2% glucose to repress TamA synthesis, harvested (2,500 g , 5 min, 4 °C) and then TamA expression was induced with 0.02% arabinose for 5 min (pulse). Cells were recovered and resuspended in media containing 0.2% glucose at room temperature to ‘chase’ the protein produced during the ‘pulse’ phase of the experiment to minimize the localization of overexpressed TamA in cytoplasmic inclusion bodies. To assay for co-immunoprecipitation of TamA and TamB, E.coli was cultured as described above and harvested (10,000 g , 15 min, 4 °C). The total membrane fraction was solubilized at a protein concentration of 1.25 mg ml −1 in 1% DDM. After centrifugation at 20,000 g for 15 min to remove insoluble material, the solubilized fraction was added to anti-TamA antibodies pre-bound to protein A Sepharose beads (Santa Cruz Biotechnology). The samples were gently rotated at 4 °C for 16 h. The resin was washed with wash buffer (0.1% DDM, 20 mM TRIS, 50 mM NaCl, pH 7.5, 1 mM phenylmethyl sulphonyl fluoride and 10% (w/v) glycerol) three times before the bound protein fraction was eluted with SDS–PAGE sample buffer. The eluted proteins were analysed by SDS–PAGE and immunoblotting with antisera recognizing TamA, TamB, BamA and BamC (see Supplementary Fig. 9 ). Surface exposure of the hexahistidine-tag introduced into a predicted extracellular loop in the carboxy terminus of TamA was assessed by immunofluorescence [38] with minor modifications: Poly- L -lysine-coated coverslips loaded with either fixed- or fixed and permeabilized cells were washed three times with PBS, incubated for 1 h in PBS containing 1% BSA to block nonspecific binding sites, and then incubated with anti-hexahistidine-tag antibody (BD Pharmingen; used at a 1:500 dilution) for 2 h. After washing three times with PBS, the coverslips were incubated for 1 h with Alexa Fluor 488 goat anti-mouse IgG (used at a 1/1,000 dilution). The coverslips were then washed three times with PBS and the samples visualized using either phase contrast or fluorescence using an Olympus Provis Ax70 microscope, with exposure times of 50 ms. Methods for BN–PAGE of native protein complexes from solubilized E. coli outer membranes, SDS–PAGE and analysis by immunoblotting have been previously published [39] . Briefly, total membrane fractions (at a protein concentration of 7 mg ml −1 ) were solubilized with 1% DDM in BN lysis buffer (20 mM imidazole-HCl pH 7.0, 50 mM NaCl, 50 mM 6-aminohexanoic acid, 1 mM EDTA, 1 mM phenylmethyl sulphonyl fluoride and 7.5% (w/v) glycerol) for 20 min at 4 °C, cleared by centrifugation at 20,000 g for 10 min, diluted 20-fold in 4.0% (w/v) Coomassie Brilliant Blue G-250 and 100 mM 6-aminohexanoic acid. Samples were analysed by electrophoresis on 4–14% gradient polyacrylamide gels. Protein production and purification In all cases, cultures of E. coli were harvested and membrane fractions subject to Ni-NTA affinity chromatography as previously described [40] . Full details of primer sequences and expression plasmid construction are available on request. Briefly, the position of the hexahistidine-tag inserted into the eighth interstrand loop (Loop 8) of TamA is documented ( Supplementary Fig. 1 ) and was achieved using Quick-change PCR with primers Forward-TamA-C-term-6xHis (5′-GTC GCG GAT AAA GAC CAC CAC CAC CAC CAC CAC GAA CAC GGG TTA CAG-3′) and Reverse-TamA-C-term-6xHis (5′-CTG TAA CCC GTG TTC GTG GTG GTG GTG GTG GTG GTC TTT ATC CGC GAC-3′). For overexpression of TamB, the coding sequence for the protein was truncated by PCR to remove the signal anchor sequence that would anchor TamB in the inner membrane. The truncated coding sequence was instead cloned into the plasmid pET22b as an in-frame fusion with the cassette encoding the leader sequence of PelB, and the modified TamB was purified from soluble periplasmic extracts of BL21(DE3) cells. The 60 kDa passenger-domain and 50 kDa barrel-domain fragments of Ag43 were expressed by cloning Forward-Ag43His8 (5′-GCC CAC AGC GTC AGC GGC CAC CAC CAC CAC CAC CAC CAC CAC AGC AGC GCT GAA GGG TAT-3′) and Reverse-Ag43His8 (5′-ATA CCC TTC AGC GCT GCT GTG GTG GTG GTG GTG GTG GTG GTG GCC GCT GAC GCT GTG GGC-3′) into the plasmid pCO2 (ref. 41 ) and the protein expressed in XL10-gold cells to overexpress Ag43 and have it accumulate in inclusion bodies. The cells were harvested, lysed with an Avestin homogeniser and centrifuged at 10,000 g for 15 min. The pellets were washed by buffer containing 0.5% (v/v) TritonX, centrifuged at 10,000 g for 10 min; repeated a total of three times. The pellets were resuspended and washed with buffer without Triton X. The pellets were then resuspended in 6 M urea and incubated over night at 4 °C. Any material that did not dissolve in urea was removed by centrifugation at 20,000 g for 20 min at 4 °C. The urea solution contained a mixture of 50, 60 and 110 kDa forms of Ag43 (110 kDa) as judged by SDS–PAGE ( Supplementary Fig. 7a ). The mixture of Ag43 forms was subject to Ni-NTA metal affinity chromatography and subsequent s200 size-exclusion chromatography, under denaturing conditions, to purify each form of Ag43. Purified, urea-denatured Ag43 was diluted 20-fold into 20 mM TRIS and 150 mM NaCl solution to a final concentration of 50 μg ml −1 protein, followed by dialysis in 20 mM TRIS and 150 mM NaCl to remove urea for 2 h at 4 °C before QCM-D or MCNR analysis. Dynamic light scattering The mean protein size and distribution were determined by dynamic light scattering (Zetasizer Malvern Instrument Ltd, UK) All measurements were carried out in triplicate at 20° after 5 min of equilibration time, in a buffer containing 20 mM TRIS, 150 mM NaCl and 0.03% DDM. Atomic force microscopy AFM measurements were performed at room temperature in solution, using the NanoWizard II AFM system at the Melbourne Centre for Nanofabrication. AFM tapping mode images were obtained using Si3N4 cantilevers (MSNL-10, cantilever D, k =0.1 N m −1 , Bruker, Santa Barbara, CA). Deflection images were simultaneously acquired; analysed with the JPK data software (JPK Instruments AG, Germany). During AFM image processing, a line was drawn and a cross-section curve composed to represent the height of sample features. Substrate modifications and protein assembly The single crystals of silicon (Si) blocks were 100 mm in diameter and 10-mm thick, and were polished on the (1 0 0) face. The Si blocks were coated with a magnetic layer consisting of a 44 Å layer of permalloy, and then with 150–200 Å layer of gold by electron beam deposition (Australian National Fabrication Facility, Australian National University). The gold-coated surface was rinsed with milli-Q water and dried under a stream of N 2 gas before use. Supplementary Fig. 2 details the modification of Ni-NTA functional group. Surface modification of Ni-NTA functional group Surface modification of the Ni-NTA functional group on the gold surface was modified according to previous protocols [42] , [43] . Supplementary Fig. 2 illustrates a three-step reaction involved in the modification of Ni-NTA group on the gold surface. First, the clean gold was exposed to a solution of 5 mM mercaptopropionic acid in isoproponal overnight ( Supplementary Fig. 2a ), followed by rinsing with isopropanol three times to remove any unbound mercaptopropionic acid and dried under a stream of nitrogen gas. After that, the dried substrate was placed into a mixture of 75 mM 1-ethyl-3-(3-dimethylaminopropyl) carbodiimide and 25 mM N-hydroxysuccinimide aqueous solution for 30 min ( Supplementary Fig. 2b ), and then washed with milli-Q water. In the final step, the self-assembled monolayer was immersed in 150 mM N α′ , N α″ -bis(carboxymethyl)- L -lysine in a 0.5 M K 2 CO 3 buffer at pH 9.8 for 3 h, which formed a carboxamide linkage ( Supplementary Fig. 2c ). Excess NTA was removed by rinsing with milli-Q water and the substrate was mounted onto a liquid cell and was placed on the QCM-D machine or neutron beamline. Protein assembly on Ni-NTA surface Before adding proteins to the cell, the NTA-modified surface was incubated with a 50 mM NiCl 2 solution to charge the carboxylate groups of NTA with Ni 2+ . Subsequently, the surface was rinsed with water and then 20 mM TRIS/150 mM NaCl/0.5% Elugent or 0.03% DDM solution, pH 7.5. Protein solutions (0.1 mg ml −1 ) of ten times the cell’s void volume were then injected using a flow pump. Detergent-solubilized TamA (in 20 mM TRIS, 150 mM NaCl and 0.03% DDM) was injected into the cell and, after protein adsorption, the surface was rinsed with the buffer without detergents before introducing a lipid bilayer. The supported bilayer was formed by POPC for QCM and 1-palmitoyl (d31)-2-oleoyl- sn -glycero-3-phosphocholine for neutron reflectometry co-adsorption with DDM with a molar ratio of 1:6 at final concentration of 1 mg ml −1 in buffer followed by further adsorption from 10 to 100 times diluted solution [19] . After equilibrium, the surface was rinsed with ten times volume of buffer without detergent to remove residual DDM. Finally, Ag43 was introduced into the flow chamber to a final concentration of 0.1 mg ml −1 . Quartz crystal microbalance with dissipation monitoring QCM-D measurements were performed using a Q-SENSE E4 system equipped with an Axial Flow Chamber, held a constant temperature at 25 °C during the experiments. The experimental setup and procedure for QCM-D have already been described elsewhere [30] , [31] , [32] . Briefly, on adsorption of matter binding to the surface of a sensor crystal; the change in frequency of the sensor movement (Δ f ) reflects the film mass (including coupled water) with a time resolution of 1 s. Magnetic contrast neutron reflection Magnetic contrast neutron reflection was carried out on the time-of-flight CRISP reflectometer at ISIS, Spallation Source (UK). The polarized beam was produced using a polarizing supermirror that transmits one neutron spin state down the beamline and reflects the other. The neutron beam then passes through guide fields to maintain the spin direction and a spin flipper that controls the final spin state (spin up or down) of neutron beam. The sample is maintained within a permanent magnetic field (~0.2 Tesla) to control the magnetization direction of the magnetic reference layer in the sample. The measurements were undertaken using a single detector at a fixed angle of θ =1.5°. The sample was measured at four angles (0.2°, 0.35°, 0.8° and 1.8°) in contact with a water solution. Reflected beam data used reduced data collection times (0.15 h for θ 1 , 0.25 h for θ 2 , 0.5 h for θ 3 and 2 h for θ 4 ) to achieve the Q range of up to 0.3 Å −1 . Direct beam measurements were collected in transmission through the Si blocks under the same collimation conditions for 1 h each. The reflectivity, R , is measured as a function of momentum transfer Q , which is defined as Q =4 π sin θ / λ , where θ is the angle of incident and λ is the neutron wavelength [44] . R ( Q ) is approximately given by ; where ρ ( Q ) is the one-dimensional Fourier transform of ρ ( z ), the SLD distribution normal to the surface. Therefore, there is a direct relation between reflectivity, R ( Q ) and the structure interface, ρ . If there are mixed layers containing two components, A and B, and water ( w ), the SLD will be ρ = φ A ρ A + φ B ρ B + φ w ρ w , where φ is the volume fraction of each layer and ρ can be different contrasts from the same layer/substance, called contrast variations. For the contrast variations, we used two different approaches. Polarized neutron can generate a magnetic contrast that is able to produce simultaneously two data sets from exactly the same layer. The advantages of using magnetic contrasts have been previously discussed [27] , [28] . We also used isotopic contrast by conducting experiments in three different buffer compositions (D 2 O, H 2 O or a mixture of D 2 O/H 2 O referred to as gold matched water). The isotopic approach is described elsewhere [33] . Data analysis The data were reduced on CRISP, and the resolution function was automatically calculated and was used in the model fitting. Analysis of the MCNR profiles was performed using MOTOFIT analysis software [45] . The software uses a conventional optical matrix method that treats the neutrons in the same way as light and applies standard optics to model the reflectivity profiles. MOTOFIT allows the variation of SLD, layer thickness and solvent content of an arbitrary number of layers and calculates the reflectivity from the optical matrix model. It is also possible to add a roughness to the layers using the Abeles method. Briefly, the layer is divided into several sublayers and then a characteristic matrix is evaluated for each sublayer, from which the whole reflectivity can be calculated exactly. The same layer with multiple data sets, with different magnetic and isotopic contrasts, is fitted simultaneously until the satisfactory fit is obtained (smallest χ 2 -value in the genetic algorithm). The best-fit model gives information about the SLD ( ρ ), thickness and roughness of each layer. When a layer is composed of just two components, a chemical species or its fragment s and water w , the SLD is given by: where ρ w and ρ s are the scattering length densities of the two components, respectively, and φ is the volume fraction of species in the layer. If more than one chemical species is present, then ρ s is determined by the volume fraction of each species in the layer. In practice, MOTOFIT allows fitting of ρ s and φ s as separate variables. If n water molecules are bound to each molecule or fragment of species a, equation (1) can be written as: where ∑ b s corresponds to neutron scattering lengths of each species, V a is the volume of monolayer fragment, b w scattering length of water and ρ layer is the SLD of the layer. Substituting V a from this equation (1− φ ) V a = nV w into equation (2). Such that: The relation between volume, V s and V w , thickness, τ , and the area per adsorbed molecule, A, is given by Substituting V s =(1− φ ) V a = φ · A · τ into equation (2), the area per adsorbed molecule may be calculated using the equation below: It is common to refer to the surface excess Γ(μmol m −2 ), which is given by: where A is the area per molecule, N a is the Avogadro’s number. These lead to the basic information of the volume fraction of solvent φ , the area per absorbed molecule A and the surface excess Γ (μmol m −2 ). All models include a 15-Å oxide layer on the surface of the silicon substrates and subsequently there are three layers of permalloy, gold and Ni-NTA on the top of oxide layer. Protein layers will assemble on the top of Ni-NTA. How to cite this article : Shen, H.-H. et al. Reconstitution of a nanomachine driving the assembly of proteins into bacterial outer membranes. Nat. Commun. 5:5078 doi: 10.1038/ncomms6078 (2014).